Pressure-stabilized lithium caesides with caesium anions beyond the −1 state Main group elements usually assume a typical oxidation state while forming compounds with other species. Group I elements are usually in the +1 state in inorganic materials. Our recent work reveals that pressure may make the inner shell 5 p electrons of Cs reactive, causing Cs to expand beyond the +1 oxidation state. Here we predict that pressure can cause large electron transfer from light alkali metals such as Li to Cs, causing Cs to become anionic with a formal charge much beyond −1. Although Li and Cs only form alloys at ambient conditions, we demonstrate that these metals form stable intermetallic Li n Cs ( n =1–5) compounds under pressures higher than 100 GPa. Once formed, these compounds exhibit interesting structural features, including capped cuboids and dimerized icosahedra. Finally, we explore the possibility of superconductivity in metastable LiCs and discuss the effect of the unusual anionic state of Cs on the transition temperature. The propensity of losing or gaining electrons is an essential trait of an element that determines its chemical reactivity and the structures and properties of the compounds formed [1] , [2] . As revealed by the atomic shell structure, the outermost atomic orbital and the respective number of electrons occupying the orbital control this fundamental feature. The atomic orbitals below and above (in energy) the outermost shell are usually not essential in defining the chemical properties, although these orbitals may still play a minor role. The main group elements on the left side of the periodic table (group I and II) tend to lose electrons in these outermost orbitals and assume a +1 or +2 oxidation state [2] . However, alkali metals may also exhibit an atypical charge state of −1 in a class of compounds called alkalides. These unusual compounds contain alkali metal anions as well as alkali cations embedded in organic molecules such as cryptands or crown ethers [3] , [4] , [5] , [6] , [7] . The unique oxidation states are related to another class of materials called electrides [6] , [8] , [9] , [10] , [11] , [12] . When electrons are detached from the embedded alkali metal cations, they either fill the interstitial sites forming electrides or, if there are alkali metal atoms available, bind loosely to them. The alkali metal anions therefore exhibit large polarizability [13] . This feature makes these anions candidates for nonlinear optics. However, no alkali metal anion with a charge beyond −1 has been reported thus far. In a recent study using first principles calculations, we demonstrated that the energy of the Cs 5 p orbitals may become higher than that of the F 2 p under pressure, and thus, Cs and F can form stable CsF n ( n >1) compounds [14] . The CsF n units are stable in the form of neutral or ionic molecules with bonding features and properties that resemble the isoelectronic XeF n . In this work, we demonstrate that pressure can lead to a new chemical inclination of Cs, which is the opposite of the above effect. We demonstrate that when mixing with light alkali elements such as Li under pressure, Cs can gain electrons and become negatively charged and form various stable intermetallic compounds with various compositions. In some of these new structures, the charge of Cs extends well beyond −1. Despite the wide range of stoichiometries, many compounds consist of similar Cs–Li polyhedrons as building blocks for their crystal structures. The structures of these compounds might be quite unusual. For example, the high-pressure structure of Li 3 Cs consists of dimerized Li icosahedra. Computational approach Our approach is based on a first principles method within the density functional theory (DFT) scheme [15] , [16] . This method can achieve very high accuracy in calculating total energies and optimizing atomic structure. This method has been successfully used in predicting numerous new materials and structures at ambient condition as well as under high pressures [17] , [18] , [19] , [20] . To search for stable Li–Cs structures with variable compositions under high pressure, we employed an effective and unbiased crystal structure searching method based on the particle swarm optimization (PSO) algorithm [21] , [22] . This method has been successfully used to predict structures of many novel compounds under pressure [23] , [24] , [25] . Our structure search included both Li-rich and Cs-rich compounds, Li n Cs m in which n =1,2,3,4,5 ( m =1) or m =1,2,3,4 ( n =1). Several structures in a previous study on alkali metal compounds [26] , including the Laves phase of MgZn 2 type, were also considered. However, none of these structures were more energetically favourable than the PSO searched structures. The results of the search for the lowest enthalpy structure as a function of the pressure for each compound are presented in Supplementary Figs 1–8 . To compare the stability of Li n Cs m compounds, we constructed a convex hull from the calculated enthalpies of the most stable structures for each composition. The enthalpy of formation per atom was calculated using the following formula: (refs 14 , 20 , 27 ). At a given pressure, the compounds located on the convex hull are stable against the decomposition into any other compositions, whereas the compounds that are above the convex hull are not energetically stable and will decompose into the compounds located on the hull. Stability of Li–Cs compounds under pressure As illustrated in Fig. 1 , Li–Cs compounds are not stable at pressures below 100 GPa. This finding is consistent with the previous knowledge that Li and Cs do not form any stable compounds under ambient conditions. However, under increasing pressure, Li 5 Cs is the first compound to become stable against decomposition into Cs and Li at approximately 70 GPa. At higher pressures, compounds with a lower Li content, such as Li 3 Cs and LiCs, become energetically more stable. Li 4 Cs is stable in a short pressure range near approximately 150 GPa. Our calculations indicate that at pressures higher than 200 GPa, Li 5 Cs may decompose into Li 3 Cs and Li or LiCs and Li. Throughout the pressure range, Li 2 Cs is not stable and can disproportionate into LiCs and Li 3 Cs. By calculating the phonon spectra, we confirmed that all of the Li n Cs compounds are also dynamically stable in their respective pressure range. Selected phonon spectra are presented in Supplementary Figs 9 and 10 . 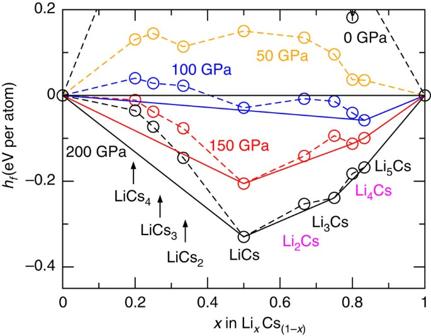Figure 1: Stability of LinCs compounds under pressure. The enthalpies of formation of LinCsm(n=1–5; m=1–4) under a series of pressures from 0 to 200 GPa. The dotted lines connect the data points, and the solid lines denote the convex hull. Details of the stable structures for Cs and Li solid can be found inSupplementary Table 1. Figure 1: Stability of Li n Cs compounds under pressure. The enthalpies of formation of Li n Cs m ( n =1–5; m=1–4) under a series of pressures from 0 to 200 GPa. The dotted lines connect the data points, and the solid lines denote the convex hull. Details of the stable structures for Cs and Li solid can be found in Supplementary Table 1 . Full size image In contrast to the Li-rich compounds, none of the Cs-rich compounds are stable in the studied pressure range. At pressures lower than 100 GPa, these compounds decompose into Li and Cs, whereas at pressures higher than 100 GPa, these compounds likely decompose into Cs and LiCs or Li-rich compounds. The tendency of decomposition of these Cs-rich compounds is also indicated by the structures found during the PSO structure search. As observed in Supplementary Fig. 11 , these structures consist of layers of LiCs and Cs. Structure features of Li-Cs compounds under pressure Despite the difference in composition and symmetry, the crystal structures of the Li n Cs compounds exhibit similarities in their local Cs–Li polyhedrons and exhibit a general evolution trend with increasing Li content. The representative structures for Li n Cs are presented in Fig. 2 . To compare the bond lengths for different stoichiometries, we chose to analyse all of the structures at 150 GPa. As observed in Fig. 2a , LiCs forms one of the simplest structures for a binary compound, the CsCl-type structure, at 150 GPa. This structure is commonly known for many ionic binary compounds. In this structure, the eight nearest neighbouring Li atoms of a Cs atom form a cube, a special hexahedron. The Cs–Li distance is 2.396 Å at 150 GPa. 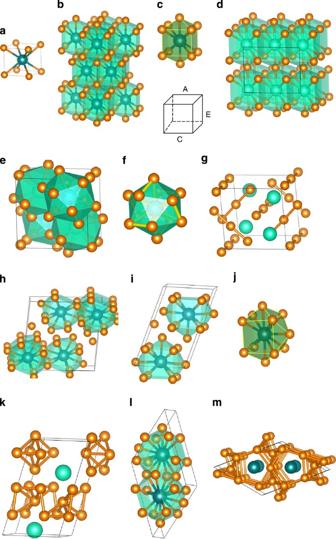Figure 2: The most stable structures of LinCs at a pressure of 150 GPa. (The parameters of all structures are listed inSupplementary Table 1). (a) LiCs in aPm-3mstructure. (b) Li2Cs in anI4/mmmstructure. (c) View of a dodecahedron. (d) Low-pressure (<100 GPa) Cmmm structure for Li3Cs. (e) Li3Cs in aPnnastructure. (f) An icosahedron with Li–Li dimers. (g) The linear Li chain in thePnnastructure of Li3Cs. (h) Li4Cs in aC2/mstructure. (i) Li5Cs in aP2/mstructure. (j) The tri-capped cube polyhedron in theC2/mstructure of Li4Cs and theP2/mstructure of Li5Cs. (k) The Li atom network in theP2/mstructure of Li5Cs. (l) The high-pressure (>150 GPa)Cmmmstructure of Li5Cs. (m) The three-dimensional Li network and the Cs atom chains in theCmmmstructure of Li5Cs. In all the structures, the large green and small tangerine balls represent the Cs and Li atoms, respectively. Figure 2: The most stable structures of Li n Cs at a pressure of 150 GPa. (The parameters of all structures are listed in Supplementary Table 1 ). ( a ) LiCs in a Pm-3m structure. ( b ) Li 2 Cs in an I4/mmm structure. ( c ) View of a dodecahedron. ( d ) Low-pressure (<100 GPa) Cmmm structure for Li 3 Cs. ( e ) Li 3 Cs in a Pnna structure. ( f ) An icosahedron with Li–Li dimers. ( g ) The linear Li chain in the Pnna structure of Li 3 Cs. ( h ) Li 4 Cs in a C2/m structure. ( i ) Li 5 Cs in a P 2/ m structure. ( j ) The tri-capped cube polyhedron in the C2/m structure of Li 4 Cs and the P2/m structure of Li 5 Cs. ( k ) The Li atom network in the P2/m structure of Li 5 Cs. ( l ) The high-pressure (>150 GPa) Cmmm structure of Li 5 Cs. ( m ) The three-dimensional Li network and the Cs atom chains in the Cmmm structure of Li 5 Cs. In all the structures, the large green and small tangerine balls represent the Cs and Li atoms, respectively. Full size image As observed in Fig. 2b , at pressures higher than 50 GPa, Li 2 Cs is stable in a structure that is identical to Au 2 Ti (ref. 28 ) and CuTi 2 (ref. 29 ); I4/mmm space group). The structure consists of face-sharing Cs–Li dodecahedrons ( Fig. 2c ), which can be viewed as adding two apices at the two opposite faces (the A and C faces in Fig. 2c ) of a cube, the original polyhedron in LiCs. The original cube is also deformed and has a shorter Li–Li distance along the direction of the apices. The corresponding c / a ratio of the cube becomes 0.87 at 150 GPa compared with the original ratio of 1 for a perfect cube. The Cs–Li distance in the deformed cube is 2.233 Å, whereas the distance of Cs to the Li atoms at the apices is 2.086 Å, which is evidently shorter. It is notable that at 0 GPa, the MnZn n -type Laves phase is observed to be 0.51 eV U −1 more stable than the P4/nmm structure (see Supplementary Fig. 5 ). However, with increasing pressure, this structure becomes less energetically favourable than P4/nmm and I4/mmm. At 50 GPa, the Laves phase is 0.57 eV U −1 higher in energy than P4/nmm. The low-pressure (<100 GPa) structure (Cmmm) of Li 3 Cs also consists of Cs–Li dodecahedrons ( Fig. 2d ). Unlike Li 2 Cs, the dodecahedrons are connected by sharing faces in the x - and y - directions and are connected by vertices in the perpendicular direction. This layered structure is not stable under higher pressure (>100 GPa) and transforms into a Pnna structure ( Fig. 2e ), increasing the coordination number of Cs from 10 to 12. The structure consists of Cs–Li icosahedrons that are slightly distorted such that every two Li atoms form dimers ( Fig. 2d ). The Cs–Li bond lengths are identical, 2.20 Å at 150 GPa. At the same pressure, the nearest Li–Li distances are 1.97 and 2.41 Å, depending on whether they are dimerized. In the whole crystal, Li forms chains with equal Li–Li distances ( Fig. 2g ). Icosahedra such as these are common in boron allotropes [30] as well as in B-rich metal borides [31] . However, the Li icosahedra observed in the Pnna structure enclose a Cs atom at their centres. The clustering of the alkali metals can be observed in alkali metal suboxides [32] and subhydrides. [33] In these compounds, the valence of the O and H atoms are maintained as −2 and −1; however, the valence of the alkali metal may vary from their typical value of +1 because the alkali metal to oxygen (or hydrogen) ratios are larger than 2:1 (or 1:1). Notably, the linear chain structure has also been observed in Li 5 H. The fundamental difference between Li–Cs and the suboxides and subhydrides is that the valence of Cs may change with different Li content. The most stable structure of Li 4 Cs under high pressure is C2/m, which consists of tricapped Cs–Li cube ( Fig. 2h ). The unique feature of Li 4 Cs is that the polyhedrons are connected by faces and form a layered structure, which is the result of the high Li concentration. Similarly, Li 5 Cs also adopts a layered structure consisting of the same tricapped Cs–Li cube ( Fig. 2i ). The structure is in space group P2/m and is most energetically favourable among all the Li 5 Cs structures from 0 to 150 GPa. Similar to dodecahedrons, the tricapped cubes can be viewed as adding three apices at the faces of a distorted cube ( Fig. 2j ), including two at the opposite faces (denoted as A and C in Fig. 2c ) and one at the side (denoted as E in Fig. 2c ). The cube is deformed. At 150 GPa, the Cs–Li distances for the four Li atoms on face E are 2.17 Å, whereas the Cs–Li length for the opposite face is 2.33 Å. The Cs–Li distances of Li atoms capped on A and C faces and of Li atoms capped on the E face are 2.19, 2.17 and 2.12 Å, respectively. The polyhedrons are connected by both sharing the face opposite to the capped side face (face E) and by sharing the two Li atoms capping the two opposite faces (A and C). The Li atoms are clustered and form two-dimensional layers in Li 5 Cs ( Fig. 2k ). At pressures higher than 150 GPa, Li 5 Cs undergoes a phase transition to a Cmmm structure ( Fig. 2l ). This structure is three dimensional, containing interatomic channels enclosed by Li atoms. Compared with the P2/m structure, the coordination number of Cs increases from 11 to 14. The Li atoms in this structure form a three-dimensional network, which contains opening channels that accommodate the Cs atomic chains ( Fig. 2m ). Electronic structures and the nature of chemical bonds To examine the nature of the chemical bonds in Li–Cs compounds and to reveal the mechanism of the formation of these compounds, we calculated the density of states (DOS) and the projected DOS (PDOS) as well as the electron localization function (ELF) of these compounds. The results are presented in Fig. 3 . As is evident by the large DOS at the Fermi level, these compounds are metallic. Notably, the states around the Fermi level show large components of Cs 5 d as well as Li 2 p , whereas the contribution from Cs 6 s and Li 2 s to the states near the Fermi level is quite small. This finding indicates a large charge transfer from the Li 2 s and Cs 6 s to the Cs 5 d and Li 2 p orbitals. Large electron transitions from s to p orbitals have been reported to occur for alkali metals under pressure. In fact, these transitions are major factors for high-pressure structural transitions in Li and Na [34] . With an increasingly Li-rich composition, the Cs 5 d contribution below the Fermi level increases (the orange line in Fig. 3d ), indicating more charge transfer into Cs 5 d states. The calculation of the 5 d occupation strongly depends on the radius of the sphere in which we perform the integration of the PDOS. We therefore define the sphere by the volume of the Bader basins, which is calculated by the stationary points of the charge density (see below). Another interesting trend of PDOS is the band dispersion of the Cs 5 p states located at approximately 5–20 eV below the Fermi level. With an increasingly Li-rich composition, the Cs 5 p states narrow and exhibit stronger isolated atomic orbital features. This finding is consistent with the Cs anions becoming more isolated in the Li matrix as the Li content increases. 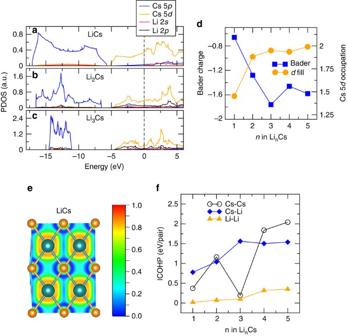Figure 3: Electronic structures and the nature of Li–Cs bonds. (a–c) The calculated projected density of states per atom (PDOS) for LiCs in the CsCl structure, Li2Cs in theI4/mmmstructure and Li3Cs in thePnnastructure. All the results were obtained at 150 GPa. The solid blue, orange, red and black lines show the contribution of the Cs 5p, Cs 5d, Li 2sand Li 2porbitals. The dashed vertical lines represent the Fermi level. (d) The Bader charge and d-band filling of LinCs (n=1–5) at 150 GPa. (e) The calculated electron localization functions of LiCs in the CsCl structure and at 150 GPa. The cutoff plane is (110). (f) The calculated integrated crystal orbital Hamiltonian populations (ICOHP) for Cs–Cs, Cs–Li and Li–Li pairs in LinCs compounds at 100 GPa. The convention of the sign is that a positive ICOHP represents bonding states. Figure 3: Electronic structures and the nature of Li–Cs bonds. ( a – c ) The calculated projected density of states per atom (PDOS) for LiCs in the CsCl structure, Li 2 Cs in the I4/mmm structure and Li 3 Cs in the Pnna structure. All the results were obtained at 150 GPa. The solid blue, orange, red and black lines show the contribution of the Cs 5 p , Cs 5 d , Li 2 s and Li 2 p orbitals. The dashed vertical lines represent the Fermi level. ( d ) The Bader charge and d-band filling of Li n Cs ( n =1–5) at 150 GPa. ( e ) The calculated electron localization functions of LiCs in the CsCl structure and at 150 GPa. The cutoff plane is (110). ( f ) The calculated integrated crystal orbital Hamiltonian populations (ICOHP) for Cs–Cs, Cs–Li and Li–Li pairs in Li n Cs compounds at 100 GPa. The convention of the sign is that a positive ICOHP represents bonding states. Full size image The charge transfer between Li and Cs atoms can be more directly illustrated using Bader’s Quantum Theory of Atom-in-Molecules approach [35] , or in short, the Bader charge. This charge is calculated by partitioning the space into Bader basins around each atom based on the stationary points of charge density. The integration of charges in each basin will give the total charge of each atom. For easy comparison, we calculated the Bader charge of each compound at 150 GPa (the blue line in Fig. 3d ). The calculated Cs Bader charges for Li n Cs ( n from 1 to 5) are −0.66, −1.28, −1.76, −1.46 and −1.58, respectively. The Bader charges indicate a large charge transfer from Li to Cs. The Cs Bader charge increases almost linearly from LiCs to Li 3 Cs (becoming more negative) and stabilizes from Li 3 Cs to Li 5 Cs. This result exhibits a similar trend with increasing Li content as the filling of Cs 5 d states ( Fig. 3d ). The results suggest that the Li and Cs form intermetallic compounds with large ionic interactions, and a large charge transfer from Li to Cs, mainly filling Cs 5 d states, is the major factor that stabilizes Li n Cs compounds. In ionic compounds, it is common that the calculated Bader charges are significantly smaller than the formal oxidation numbers. For example, in CsF, the Bader charge of Cs is only 0.81 e (ref. 14 ). Although we cannot absolutely assign the formal oxidation state for Cs in Li n Cs compounds using this method, the calculated Bader charges suggest that the oxidation state is potentially beyond −2 for Cs in Li n Cs ( n >2) compounds. The ELF maps the probability of finding electron pairs in different areas of the crystal [36] , [37] . The larger ELF values (>0.5) indicate the formation of covalent bonds. The calculated ELF of LiCs at 150 GPa is shown in Fig. 3e . The largest ELF values are observed near the Cs and the Li atoms, corresponding to the core 5 p electrons in Cs and 1 s electrons in Li. Between Li and Cs atoms, there are large areas with very small ELF values, which is typical for ionic and metallic bonding [38] . Furthermore, there are areas between Cs atoms with large values of ELF (approximately 0.34). Although this ELF value does not correspond to strong covalent bonds, it does indicate a large covalent bonding component between the neighbouring Cs atoms. In fact, a similar value of ELF was observed for Au(CN) 2 − , in which Au–C was observed to be covalently bonded according to both computational and experimental evidence 39 . Because the bonding between Cs and Li atoms in Li n Cs compounds is considerable, we examine these interactions by also calculating the crystal orbital Hamilton populations and the respective integrated crystal orbital Hamilton populations (ICOHPs) [40] using the linear muffin-tin orbital (LMTO) method. The ICOHP counts the energy-weighted population of wavefunctions between two atomic orbitals for a pair of selected atoms; therefore, this value tends to scale with bond strength (metallic or covalent) in compounds [40] . As shown in Fig. 3f , the values of the ICOHP between the pairs Cs–Cs and Cs–Li are quite large for LiCs and become even more significant with increasing Li composition, indicating that the Cs–Cs and Cs–Li bonds become stronger. The ICOHP of Cs–Cs and Cs–Li can be as large as 2.042 and 1.539 eV per pair, respectively, in Li 5 Cs. In comparison, the ICOHP of Cs–F in CsF 3 at 100 GPa is 1.787 eV per pair [14] . The large variation of Li 3 Cs from the general trend of ICOHPs is most likely caused by the fact that Cs atoms are enclosed in Li icosahedra, and therefore, Cs–Cs bonding is weakened. The Li–Li ICOHPs are much smaller (close to zero) in LiCs, Li 2 Cs and Li 3 Cs but become considerably large in Li 4 Cs and Li 5 Cs, which is a result of Li clustering. The decomposition of ICOHP into atomic orbitals indicates that the major contributions for Cs–Cs pairs are between the Cs 5 p and 5 d orbitals. For example, the Cs–Cs ICOHP for LiCs at 100 GPa is 0.372 eV per pair, and its major contributions come from 6 s -5 p , 6 s -6 p , 5 p -5 p and 5 p -5 d , corresponding to decomposed ICOHP values of −0.267, 0.269, −0.305 and 0.612 eV per pair, respectively. Superconductivity Noticing that both Li and Cs can become superconducting under compression [41] , [42] , [43] , [44] , we examined the electron phonon coupling and superconducting transition for the LiCs compound. 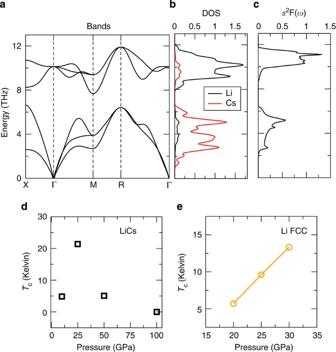Figure 4: Phonon spectrum and superconductivity of LiCs. (a) The calculated phonon spectrum of the LiCs crystal at 50 GPa. (b) The calculated projected phonon density of states (PDOS) of LiCs at 50 GPa into Li (black line) and Cs (red line) contributions. (c) The calculated Eliahsberg electron-phonon spectral densityα2F(ω) of LiCs. (d) The calculated value of the superconducting transition critical point (Tc) for LiCs as a function of the pressure. (e) The calculated value ofTcfor Li in a face-centre cubic (FCC) structure as a function of the pressure. Figure 4a,b shows the phonon bands and partial density of states of LiCs in a CsCl structure at 50 GPa. At this pressure, LiCs is metastable and can in principle decompose into Li and Cs. However, as revealed by the phonon spectra, the structure is dynamically stable. We find that the dynamic stability remains for LiCs under pressures as low as 10 GPa. Therefore, if the temperature is low enough, the LiCs can maintain the CsCl structure at much lower pressure. The phonon bands consist of well-separated low- and high-frequency branches. The components of the low- and high-frequency branches are dominantly Cs and Li vibrations, respectively. Figure 4: Phonon spectrum and superconductivity of LiCs. ( a ) The calculated phonon spectrum of the LiCs crystal at 50 GPa. ( b ) The calculated projected phonon density of states (PDOS) of LiCs at 50 GPa into Li (black line) and Cs (red line) contributions. ( c ) The calculated Eliahsberg electron-phonon spectral density α 2 F ( ω ) of LiCs. ( d ) The calculated value of the superconducting transition critical point ( T c ) for LiCs as a function of the pressure. ( e ) The calculated value of T c for Li in a face-centre cubic (FCC) structure as a function of the pressure. Full size image Figure 4c displays the calculated Eliashberg spectral function, which peaks in both low-frequency and high-frequency regions, corresponding to the low- and high-frequency Cs and Li vibrations. This feature indicates that both Cs and Li vibrations contribute to the superconductivity. However, although calculating the electron-phonon coupling constant λ , the spectral function is weighted by the inversion of its frequency; therefore, the contribution of high-frequency branches dominated by Li vibration modes is not as great as that observed in Fig. 4c . At 50 GPa, the electron-phonon coupling constant λ is calculated to be 0.65, and the logarithmic average frequency is 294 K. Applying the above electron-phonon coupling results in the McMillan-Allen-Dynes equation [45] , [46] . , we find a T c of 5.07 K for LiCs in the CsCl structure at 50 GPa. A typical value of 0.15 is used for the Coulomb pseudopotential μ *. We also find that T c has a significant dependence on pressure ( Fig. 4d ). The highest T c among the pressure points that we examined was observed at 25 GPa and is as high as 21.4 K. At 10 GPa, the T c is 4.9 K. A similar reduction of T c occurs by increasing the pressure. At 100 GPa, there is no superconducting transition for LiCs. To validate this approach, we also calculated the electron-phonon coupling constants and transition temperatures for Li and Cs in the face-centred cubic (FCC) structure under pressure. The results for Li are presented in Fig. 4e . Our results compare well with experimental measurements [46] , [47] and previous density functional calculations [48] . For example, T c is calculated to be 5.71 and 13.32 K for 20 and 30 GPa, respectively, compared with the values of 5.47 K for 20.3 and 30 GPa measured by Deemyad et al . [46] . The T c for FCC Cs at 5 GPa is calculated to be 5.29 K. A previous work based on DFT calculations observed that T c of FCC Cs increases with increasing pressure [49] . Although the pressure in that work is below 4 GPa, the extrapolation of their results to 5 GPa and to a μ * value of 0.15 will roughly yield a T c value of approximately 6 K ( Supplementary Fig. 8 in ref. 50 ). We also find that T c increases with increasing pressure. At 10 GPa, T c is 13.61 K, as observed by our calculation. The superconducting transition in Cs metal under pressure is associated with the transfer of electrons from 6 s to 5 d orbitals [41] . Such a s – d transition makes Cs behave like a 5 d transition metal and possess stronger electron-phonon coupling. The Li component in LiCs has two effects. The first effect is to increase the density of 5 d electrons because of the transfer of electrons from Li 2 s to Cs 5 d . Furthermore, the strong coupling of the electrons with the Li vibrations that dominate the high-frequency phonon spectra may also enhance T c , although the eventual T c may not be as high as that in Li under the same pressure. The underlying formation mechanism of stable Li–Cs compounds under pressure is the energy reordering of atomic orbitals. Under ambient condition, the Cs 5 d orbitals are higher in energy than the Cs 6 s orbitals, which in turn are similar to those of Li 2 s . When mixing the two elements, only alloys can form and not stoichiometric compounds because of the similarity of the atomic orbital energies. However, owing to the smaller size, Cs 5 d orbitals are less affected by pressure-induced volume reduction, and their energy increases less than that of the Li 2 s orbital. Under high enough pressure, the charge transfer from Li 2 s to Cs 5 d will reduce the total energy enough to stabilize the Li n Cs ( n >1) compounds. The effect of this orbital reordering under pressure in compressed alkali metals has already been reported in the literature. In a previous work, a large charge transfer from 4 s to 3 d was observed for K under high pressure. Because of that, K behaved like a transition metal under those conditions [50] . A similar phenomenon has also been observed for Cs [51] . In contrast, the charge transfer between two different alkali metals due to energy reordering of s and d orbitals and the possibility of forming compounds between these metals has not been examined before. Hafner speculated on the possibility that s – d hybridization could stabilize alkali metal compounds while studying the presence of a Laves phase of Na 2 Cs at ambient condition [26] . However, our calculations find that the 5 d filling of Na 2 Cs is only 0.03. Furthermore, the Bader analysis reveals a transfer of electrons from Cs to Na, indicating that the electronic structure of the Na 2 Cs Laves phase is significantly different from the high-pressure phases of Li–Cs presented here. Considering that the energy shift of s and d orbitals under pressure is a general trend, this phenomenon should not be limited to the Li–Cs system. In fact, we have observed in other calculations the formation of stable Li–Xe and Mg–Xe intermetallic compounds, in which Xe atoms gain electrons from Li or Mg and form negatively charged ions. Furthermore, we emphasize that although the Cs anions (and other alkali metal anions) have previously been observed in organometallic molecules and compounds, their chemistry is very different from that of Li–Cs compounds: the charge on those Cs and other alkali metal anions is due to the extra occupation of the outmost s orbital instead of atomic orbital reordering and never extends beyond −1. In summary, we have demonstrated using first principles calculations and an unbiased automatic structure search technique that Cs can gain electrons and form intermetallic compounds with Li under high pressure. The underlying mechanism of this unusual bonding is the energy reordering of the atomic orbitals under pressure. The large charge transfer from Li to Cs stabilized Cs in a negatively charged state, leading to unusual features in their compounds. This phenomenon may also be observed for other elements containing unoccupied d orbitals, which would lead to the formation of anions in a priori cationic elements. Structure search To obtain stable structures for Li n Cs, we conducted an unbiased structure prediction based on the PSO algorithm as implemented in Crystal structure AnaLYsis by Particle Swarm Optimization [21] , [22] . The structure predictions were performed using a unit cell containing up to 4 Li n Cs m units at pressures ranging from 0 to 200 GPa. Electronic structure calculation The underlying ab initio structural relaxations and the electronic band-structure calculations were performed within the framework of DFT as implemented by the VASP (Vienna Ab initio Simulation Package) code [52] . The generalized gradient approximation within the framework of Perdew–Burke–Ernzerhof [53] was used for the exchange-correlation functional, and the projector augmented wave (PAW) potentials [54] , [55] were used to describe the ionic potentials. In the PAW potential for Cs, the 5 s , 5 p and 6 s orbitals were included in the valence. The accuracy of the PAW potentials were tested and compared with a full-potential method. A comparison of the equation of states ( V – P ) for LiCs calculated using PAW and a full-potential method is presented in Supplementary Fig. 12 . The cutoff energy for the expansion of the wave function into plane waves was set at 450 eV, and Monkhorst-Pack k meshes were selected to ensure that all the enthalpy calculations converged to better than 1 meV per atom. The ELF was also calculated using VASP. As implemented in VASP, ELF ranges from 0 (free electron gas) to 1 (localized electrons). Phonon spectra calculation The phonons and superconducting transition temperatures of LiCs, Li and Cs were calculated using the full-potential linear augmented plane wave method as implemented in the ELK programme ( http://elk.sourceforge.net/ ). A k -mesh of 24 × 24 × 24 was used while calculating the electron-phonon coupling matrix elements. The ICOHP was calculated using the Stuttgart version of the tight-binding LMTOs, atomic sphere approximation (TB-LMTO-ASA) programme ( http://www2.fkf.mpg.de/andersen/LMTODOC/LMTODOC.html ). How to cite this article: Botana, J. & Miao, M.-S. Pressure-stabilized lithium caesides with caesium anions beyond the −1 state. Nat. Commun. 5:4861 doi: 10.1038/ncomms5861 (2014).